Synchronization of spin Hall nano-oscillators to external microwave signals Recently, a novel type of spin-torque nano-oscillators driven by pure spin current generated via the spin Hall effect was demonstrated. Here we report the study of the effects of external microwave signals on these oscillators. Our results show that they can be efficiently synchronized by applying a microwave signal at approximately twice the frequency of the auto-oscillation, which opens additional possibilities for the development of novel spintronic devices. We find that the synchronization exhibits a threshold determined by magnetic fluctuations pumped above their thermal level by the spin current, and is significantly influenced by the nonlinear self-localized nature of the auto-oscillatory mode. With the experimental demonstration of the generation of pure spin currents—directional flows of angular momentum not tied to the flow of electrical charge—the development of spin-based electronic (spintronic) devices has entered a new phase [1] , [2] . It has now become possible to exploit a range of both electrically conducting and insulating magnetic materials that would be incompatible with conventional magnetic multilayer structures using spin-polarized charge currents. Moreover, planar device geometries operating via spin currents generated by the spin Hall effect (SHE) are generally scalable, enabling us to envision the operation of devices with dimensions ranging from nanometres to millimetres [3] , [4] , [5] , [6] , [7] , [8] , [9] , [10] , [11] . Following the pioneering work demonstrating the possibility of reducing effective magnetic damping using spin currents generated by SHE [3] , complete compensation of damping has recently been realized in magnetic nanostructures [9] , [10] , [11] . The resulting spontaneous microwave-frequency oscillations can be utilized for the generation of signals for next-generation integrated electronics. Spin-torque nano-oscillators (STNOs) driven by SHE, known as spin Hall nano oscillators (SHNOs), have several advantages over conventional STNOs. In particular, pure spin currents are less likely to cause damage by electromigration or by Ohmic heating in the ferromagnets. In addition, their geometry facilitates direct optical access to the active device area enabling unprecedented measurements by advanced magneto-optical techniques and thus elucidating the dynamic phenomena induced by spin currents [7] , [10] . One of the distinguishing characteristics of STNOs is a strong nonlinearity, which enables their efficient synchronization to external periodic signals over a wide frequency range [12] , [13] , [14] , [15] , [16] . This synchronization may allow the development of microwave sources with improved generation coherence using mutually synchronized STNO arrays. The implementation of such arrays with SHNOs is significantly more straightforward than with conventional STNOs because of their more simple, planar geometry. However, synchronization of SHNOs to microwave signals has yet to be demonstrated. Here, we report an experimental study of the response of SHNOs to external microwave signals. We demonstrate that SHNOs exhibit efficient parametric synchronization when the external driving frequency is close to twice their oscillation frequency, with a relatively wide synchronization frequency interval controlled by the magnitude of the microwave signal and by the dc current flowing through the device. In contrast with the synchronization of conventional STNOs based on giant magnetoresistive structures [15] , [16] , the synchronization of SHNOs occurs only above a certain threshold external microwave signal power. Our analysis shows that synchronization is suppressed below the threshold through the influence of spin wave modes enhanced by the spin current. Sample characteristics Our test devices are formed from a bilayer comprising a 8-nm-thick film of Pt and a 5-nm-thick film of Permalloy (Py) patterned into a disk with the diameter of 4 μm ( Fig. 1a ). Two 150-nm-thick Au electrodes placed on top of the bilayer form an in-plane point contact. The endpoints of the Au electrodes have a 50-nm radius and are separated by a 100-nm wide gap. To induce oscillations of the Py magnetization, a dc current I is applied between the Au electrodes. Calculations of the current distribution based on a three-dimensional model of the device show that, because of the large difference between the sheet resistances of the electrodes and the Py/Pt bilayer, the current is concentrated predominantly in the gap between the electrodes within an area with a characteristic size of about 250 nm ( Fig. 1b ). 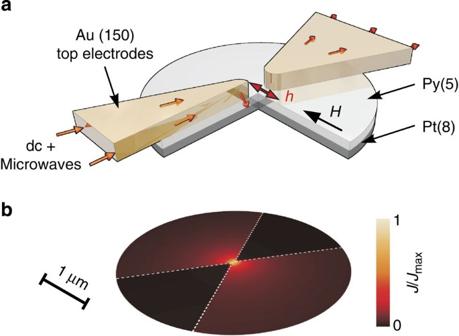Figure 1: Experimental configuration. (a) Schematic of the test device. (b) Normalized calculated distribution of the driving current density in the device plane. Figure 1: Experimental configuration. ( a ) Schematic of the test device. ( b ) Normalized calculated distribution of the driving current density in the device plane. Full size image The electric current flowing in the Pt layer produces, via the SHE, a pure spin current directed perpendicular to the bilayer plane [17] , [18] . This spin current exerts a spin-transfer torque on the magnetization of the Py, which results in a modification of its dynamic magnetic damping [3] , and an enhancement (or suppression) of thermal magnetization fluctuations [7] depending on the direction of the electric current relative to the magnetic field H . In the studied geometry, positive current as defined in Fig. 1a results in reduction of the effective damping. The magnetization of Py starts to auto-oscillate when the dynamic damping is completely compensated [9] , [10] , [11] . The magnetization dynamics in the Py layer was detected by micro-focus Brilloin light scattering spectroscopy (BLS) [19] . The BLS intensity at a given frequency is proportional to the intensity of magnetization oscillations at this frequency at the position of the probing laser spot, which in our experiment was centred in the gap between the electrodes. 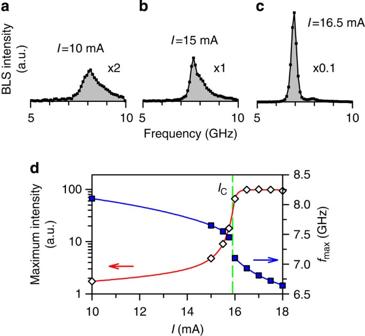Figure 2: Evolution of the spectra under the influence of current. (a–c) Magnetization oscillation spectra recorded at the labelled values of dc current. (d) Maximum BLS intensity (open symbols) and the corresponding frequency (solid symbols) versus current, atH=800 Oe. Lines are guides for the eye. The data were obtained by BLS. Figure 2 illustrates the evolution of the BLS spectra under the influence of current I , at H =800 Oe. A broad peak observed at I <16 mA is caused by thermal magnetization fluctuations enhanced by the spin current [7] , [8] , [9] , [10] , as illustrated for I =10 mA and 15 mA in Fig. 2a,b , respectively. A narrow peak with the center frequency of about 7 GHz appears below the thermal fluctuation peak at I =15.75 mA, then quickly increases in amplitude around I =16 mA, and saturates at I >16.5 mA ( Fig. 2c ). We identify the range 15.75 mA< I <16 mA with the metastable auto-oscillation regime stimulated by thermal effects, and the value I =16 mA with the critical current I C at which the dynamical damping is completely compensated by the spin current, resulting in the onset of stable auto-oscillation. This interpretation is supported by the analysis of the dependence of spectral characteristics on current, Fig. 2d . The maximum detected BLS intensity gradually increases with increasing I<I C , abruptly jumps at I = I C , and then saturates at I >16.5 mA (note the logarithmic scale on the corresponding vertical axis in Fig. 2d ). Meanwhile, the frequency f max corresponding to the maximum of the BLS intensity gradually decreases with increasing I<I C due to the nonlinear frequency shift associated with the enhancement of thermal magnetization fluctuations, and then drops abruptly at I = I C . This abrupt decrease clearly marks the onset of auto-oscillations via the formation of a nonlinear self-localized spin-wave ‘bullet’ mode [10] , [11] , [20] at frequency below the linear spectrum of propagating spin waves. The transition to the auto-oscillation regime is observed only at I >0, while at I <0 thermal magnetization fluctuations are increasingly suppressed and no auto-oscillation is observed. Rotation of the static field by 180° results in the inversion of these effects with respect to the direction of I , in agreement with the symmetry of the SHE [17] , [18] . Figure 2: Evolution of the spectra under the influence of current. ( a – c ) Magnetization oscillation spectra recorded at the labelled values of dc current. ( d ) Maximum BLS intensity (open symbols) and the corresponding frequency (solid symbols) versus current, at H =800 Oe. Lines are guides for the eye. The data were obtained by BLS. Full size image Effects of the external microwave signals To study the effects of external signals on the oscillation characteristics of our SHNOs, we used a bias tee to apply a microwave current at frequency f MW simultaneously with the dc current I . The microwave current induces in the Py film a dynamic Oersted magnetic field h ( Fig. 1a ). The maximum power of the applied microwave signal was P =2 mW, which corresponds to a dynamic field h ≈57 Oe. The spatial in-plane distribution of h was found to be very close to that of the sheet current density ( Fig. 1b ). We note that the operation of SHNO is optimized when H is perpendicular to the current flow, such that h || H . In this geometry, the dynamic magnetic field couples to the dynamic magnetization through the parametric process that becomes efficient when the driving frequency is close to twice the auto-oscillation frequency [21] , [22] . By rotating H away from this direction, one can in principle achieve direct linear coupling of magnetization to external microwaves at the fundamental frequency. However, because of the symmetry of SHE, such rotation results in a dramatic increase of the critical current I C (ref. 10 ), making the operation of SHNO inefficient. Therefore, we focus below on measurements with h || H , and microwave signals applied at frequencies f MW close to 14 GHz. We note that the oscillating spin-transfer torque generated by the microwave current produces an additional contribution to the parametric process. However, numerical simulations show that this contribution in our experiment is small compared with the effect of the dynamic magnetic field. First, we analyse the effects of the microwave signal at dc currents below the onset of auto-oscillation, as illustrated in Fig. 3a for I =15 mA and f MW varying from 12 to 16 GHz. The effect is significant only over a narrow frequency interval, when f MW /2 is close to the ferromagnetic resonance frequency of the Py film. A strong increase of the BLS intensity within this interval is caused by parametric spin-wave instability [23] induced by the microwave signal. 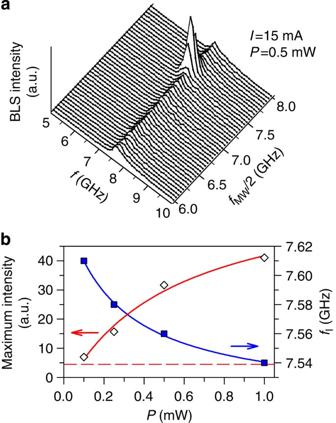Figure 3: Effects of the microwave signal below the onset of auto-oscillation. (a) BLS spectra recorded atI=15 mA, with the frequencyfMWof the microwave signal varying from 12 to 16 GHz in 0.1 GHz increments. The power of the signal isP=0.5 mW. (b) Maximum intensity of the BLS spectrum (open symbols) and the corresponding frequencyfI(solid symbols) versus driving microwave signal powerP. Solid lines are guides for the eye. Dashed horizontal line in (b) shows the maximum intensity in the absence of the microwave signal. The data were obtained by BLS. Figure 3: Effects of the microwave signal below the onset of auto-oscillation. ( a ) BLS spectra recorded at I =15 mA, with the frequency f MW of the microwave signal varying from 12 to 16 GHz in 0.1 GHz increments. The power of the signal is P =0.5 mW. ( b ) Maximum intensity of the BLS spectrum (open symbols) and the corresponding frequency f I (solid symbols) versus driving microwave signal power P . Solid lines are guides for the eye. Dashed horizontal line in ( b ) shows the maximum intensity in the absence of the microwave signal. The data were obtained by BLS. Full size image To quantify the parametric instability, we determined the frequency f I at which the peak BLS intensity reaches a maximum, at a given excitation power P . Figure 3b shows that f I monotonically decreases with increasing P , due to nonlinear frequency shift, while the corresponding maximum peak intensity exhibits a monotonic increase, gradually saturating at large P . The maximum intensity exceeds the thermal level, shown with a horizontal dashed line, only at driving powers above the threshold value ≈0.07 mW, in agreement with the theory of the parametric instability. Next, we studied the effects of the external microwave signal in the stable auto-oscillation regime of the SHNO, at I > I C . 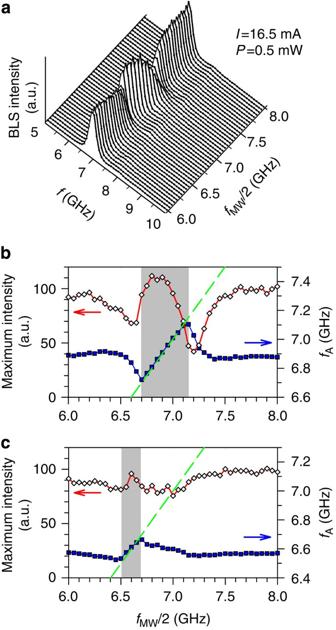Figure 4: Effects of the microwave signal above the onset of auto-oscillation. (a) BLS spectra recorded atI=16.5 mA, with the frequencyfMWof the microwave signal varying from 12 to 16 GHz in 0.1 GHz increments. The power of the signal isP=0.5 mW. (b) Maximum intensity of the BLS spectrum (open symbols) and the corresponding auto-oscillation frequencyfA(solid symbols) versus driving microwave frequency. Shaded area marks the synchronization interval. Dashed line shows the dependencefA=fMW/2. (c) Same as (b), forI=18 mA. The data were obtained by BLS. Figure 4a shows the data obtained at I =16.5 mA, in the stable auto-oscillation regime of SHNO with a saturated intensity (see Fig. 2d ). In contrast to the subcritical regime, the BLS spectra exhibit a narrow intense auto-oscillation peak, regardless of the external microwave frequency ( Fig. 4a ). When f MW /2 approaches the auto-oscillation frequency, the latter starts to exactly follow f MW /2 (solid symbols in Fig. 4b ), as expected for parametrically synchronized oscillation, and as previously observed for conventional STNOs [15] , [16] . However, unlike in conventional STNOs, where a large increase of intensity is observed in the synchronized regime [15] , the intensity of oscillation of the SHNOs varies only slightly throughout the external frequency range, with the largest intensity near the middle of the synchronization interval, and two minima near the synchronization limits (open symbols in Fig. 4b ). These behaviours persist at larger driving dc currents ( Fig. 4c ), although the width of the synchronization interval becomes noticeably reduced due to the increased magnetic noise, as discussed below. Figure 4: Effects of the microwave signal above the onset of auto-oscillation. ( a ) BLS spectra recorded at I =16.5 mA, with the frequency f MW of the microwave signal varying from 12 to 16 GHz in 0.1 GHz increments. The power of the signal is P =0.5 mW. ( b ) Maximum intensity of the BLS spectrum (open symbols) and the corresponding auto-oscillation frequency f A (solid symbols) versus driving microwave frequency. Shaded area marks the synchronization interval. Dashed line shows the dependence f A = f MW /2. ( c ) Same as ( b ), for I =18 mA. The data were obtained by BLS. Full size image Besides frequency locking demonstrated by the BLS measurements, reduction of the auto-oscillation linewidth in the synchronized regime is an important signature of synchronization. Since the BLS technique has a limited spectral resolution, we performed additional electronic spectroscopy measurements. These measurements demonstrate that the linewidth of the auto-oscillation is reduced by up to four orders of magnitude in the synchronized regime ( Fig. 5 and Supplementary Fig. 1 ). 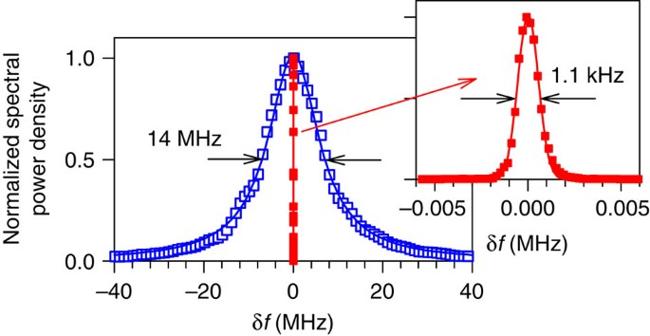Figure 5: Electronic characterization of the auto-oscillation linewidth. Spectra of SHNO auto-oscillations obtained for the free-running oscillation without external microwave signal (open symbols) and oscillation synchronized with the external microwave signal (solid symbols). Inset shows the synchronized spectrum on a finer frequency scale. δfdenotes detuning fromfMW/2. Curves show the result of the fitting of the experimental data by the Lorentzian function for the free-running spectrum, and Gaussian for the synchronized spectrum. Figure 5: Electronic characterization of the auto-oscillation linewidth. Spectra of SHNO auto-oscillations obtained for the free-running oscillation without external microwave signal (open symbols) and oscillation synchronized with the external microwave signal (solid symbols). Inset shows the synchronized spectrum on a finer frequency scale. δ f denotes detuning from f MW /2. Curves show the result of the fitting of the experimental data by the Lorentzian function for the free-running spectrum, and Gaussian for the synchronized spectrum. Full size image To gain further insight into the synchronization process, we measured the dependence of the synchronization interval Δ f S on the dynamic microwave magnetic field h , which is proportional to the square root of the driving microwave power P . The dependencies of Δ f S on P 1/2 obtained at different values of dc current are shown by the symbols in Fig. 6a . No synchronization was observed at microwave powers below ≈0.03 mW, regardless of the dc current value. At a current I =18 mA significantly above the oscillation onset, Δ f S exhibits an approximately linear dependence on P 1/2 above the threshold (circles and solid straight line in Fig. 6a ), while at smaller currents close to the oscillation onset, a rapid increase of Δ f S at small microwave power is followed by saturation (squares and diamonds in Fig. 6a ). 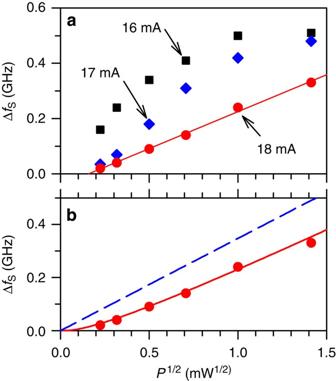Figure 6: Dependence of the synchronization interval on the dynamic field. (a) Measured synchronization interval versusP1/2, at the labelled values of dc currentI. Solid line is a linear fit of theI=18 mA data. (b) Symbols: measured synchronization interval versusP1/2, atI=18 mA. Solid curve: calculated synchronization interval in the presence of noise. Dashed curve is the same dependence calculated in the absence of noise. The experimental data were obtained by BLS. Figure 6: Dependence of the synchronization interval on the dynamic field. ( a ) Measured synchronization interval versus P 1/2 , at the labelled values of dc current I . Solid line is a linear fit of the I =18 mA data. ( b ) Symbols: measured synchronization interval versus P 1/2 , at I =18 mA. Solid curve: calculated synchronization interval in the presence of noise. Dashed curve is the same dependence calculated in the absence of noise. The experimental data were obtained by BLS. Full size image The observed behaviours are not described by the theory of synchronization of nonlinear single-mode oscillators [14] , which predicts a universally linear dependence of Δ f S on P 1/2 . The predicted dependence also starts at the origin, since the synchronization is known to be a non-threshold phenomenon. We note that the synchronization of conventional STNOs based on GMR structures was found to be generally consistent with this theory [13] , [15] , [16] . We now show that the observed synchronization threshold can be explained by the effects of thermal noise enhanced by the spin current on the self-localized ‘bullet’ oscillation mode. We base our analysis on the theory of auto-oscillator synchronization developed in Slavin and Tiberkevich [14] , applying it to the ‘bullet’ oscillation mode of the SHNOs [20] , and analytically taking into account the effect of thermal noise that was introduced numerically in Georges et al. [13] (see the Supplementary Note 1 for details). The spin-wave ‘bullet’ can be described by a perturbed nonlinear two-dimensional Schrödinger equation [20] : where, a=|a| exp[ iψ ( t )] is the complex amplitude of the ‘bullet’ mode, f 0 is the ferromagnetic resonance frequency, D is the spin-wave dispersion coefficient and N is the nonlinear frequency shift coefficient. The term F ( a , t )= F d ( a , t )+ S n ( t ) in the right-hand side of Equation (1) comprises a deterministic term F d ( a , t ) and a stochastic term S n ( t ). The former accounts for the Gilbert damping, the negative damping produced by the spin current via the spin torque mechanism, and for the Zeeman torque exerted by the external microwave signal. The stochastic term S n ( t ) describes the effect of thermal noise. For a well-developed spin-wave ‘bullet’ (dc current sufficiently above I C ) the effects of perturbations can be analysed in the framework of the modulation theory [24] . To describe the synchronization process, it is convenient to renormalize oscillation phase Φ( t )=2 ψ ( t )−2 π f MW t +ΔΦ, where ΔΦ is a nonlinear phase shift that accounts for the dependence of the generation frequency f g on the auto-oscillation amplitude a . The evolution of the renormalized phase can be then described by where, Δ f MW = f g − f MW /2, and Δ f 0 is the synchronization interval in the absence of noise, which is proportional to the amplitude h of the microwave signal, s n ( t ) is the normalized thermal white noise characterized by auto-correlation = δ ( t − t ′), and μ =(1+ v 2 )Γ( k B T / E ) is the amplitude of thermal noise measured in units of angular frequency and numerically equal to the generation linewidth of the free-running auto-oscillator. Here v is the nonlinearity coefficient, Γ is the Gilbert damping rate, k B is the Boltzmann constant, T is temperature and E is the energy of the ‘bullet’ mode that can be found using Equation (77) in Slavin and Tiberkevich [14] and Equations (6), (7) and (10) in Slavin and Tiberkevich [20] . Using the standard Fokker–Planck formalism [24] , the stochastic Equation (2) can be transformed into a deterministic Fokker–Planck-type equation for the probability distribution of the normalized phase. Solving this equation, we obtain an explicit expression for the frequency f A of the perturbed ‘bullet’ in the presence of noise where C = dΦ′ and u (Φ) =(4 π Δ f MW +2 π Δ f 0 cosΦ)/ μ . Equation (3) is the analytical solution of the synchronization problem in the presence of noise, which allows one to directly calculate the dependence of the synchronization interval Δ f S on the microwave power P . It is reduced to Equation (55) in Slavin and Tiberkevich [14] in the limit of negligible noise, μ →0. Solid curve in Fig. 6b shows the result of the calculation for I =18 mA using μ /2π=46 MHz and Δ f 0 = BP 1/2 with B= 350 MHz/(mW) 1/2 as the only fitting parameters. The inclusion of the effects of noise in the model results in a decrease of the synchronization interval Δ f S and a non-zero apparent power threshold of the synchronization process. In contrast, the same calculation neglecting the effects of noise (dashed curve in Fig. 6b ) yields no threshold for synchronization, in a qualitative disagreement with the data. The effective noise amplitude μ at room temperature can be calculated from Equation (4) with a value v ≈2 typical for the in-plane magnetized film [25] , giving μ /2 π ≈0.4 MHz (see Supplementary Note 2 ), which is significantly smaller than the value μ /2 π =46 MHz obtained by fitting the experimental data. The discrepancy between these values can be attributed to the effect of the spin current on the magnetic noise in the SHNOs: the dynamic magnetic modes are pumped to well above their thermal levels by the spin current [7] , [10] and accordingly the effective temperature of the magnetic system corresponding to the low-energy fluctuations significantly exceeds that of the lattice, resulting in a large apparent threshold for synchronization ( Fig. 6 ). To verify this hypothesis, we performed additional electronic measurements of synchronization at T =6 K. These measurements clearly demonstrate that the synchronization threshold is not reduced at cryogenic temperatures (see Supplementary Fig. 2 ), indicating that magnetic noise is dominated by the effects of spin current. We note that our analysis of the well-developed ‘bullet’ synchronization cannot quantitatively describe the dependence of Δ f S on P 1/2 obtained at dc currents close to I C (see I =16 and 17 mA data in Fig. 6a ). We can identify two mechanisms responsible for this disagreement. First, the mode rigidity assumption underlying our analysis does not hold for small oscillation amplitudes, since external perturbations can make a significant contribution to the energy balance of the ‘bullet’ mode. Second, the approximation of uncorrelated white noise is not valid in this regime as the non-equilibrium populations of magnetic modes deviate significantly from the thermal distribution in the vicinity of the damping compensation point [7] . On the other hand, at larger currents one can expect that stronger nonlinear effects result in more efficient thermalization of spin waves. In summary, we demonstrate that spin-Hall nano-oscillators can efficiently synchronize to external microwave signals, providing a route the optimization of high-frequency spintronic devices for future-generation microelectronic circuits. Since the geometry of spin Hall oscillators facilitates direct optical access to the active device area they present an unprecedented opportunity for fundamental studies of nonlinear dynamic phenomena in nanoscale systems. In addition, our results elucidate the general effects of thermal noise on the synchronization characteristics of STNOs, which may explain some of the recent observations in structures based on magnetic tunnel junctions [26] . Sample fabrication Bilayers consisting of an 8-nm-thick Pt and a 5-nm-thick Py layer were sputtered at room temperature on sapphire substrates, and coated with a 3-nm thick protective SiO 2 layer without breaking the vacuum. The bilayer was patterned into a 4 μm disk by e-beam lithography. Two pointed 150-nm-thick Au electrodes separated by a 100 nm gap were defined by e-beam lithography. The electrodes were deposited by sputtering after the protective SiO 2 layer was removed from the area of electrodes by Ar ion milling. Finally, the entire structure was coated by a 50-nm-thick SiO 2 layer to prevent oxidation. Magneto-optical measurements Micro-focus BLS measurements were performed at room temperature by focusing light produced by a continuous-wave single-frequency laser operating at the wavelength of 532 nm into a diffraction-limited spot. The light scattered from magnetic oscillations was analysed by a six-pass Fabry-Perot interferometer TFP-1 (JRS Scientific Instruments, Switzerland) to obtain information about the BLS intensity proportional to the square of the amplitude of the dynamic magnetization at the location of the probing spot. Low-temperature electronic measurements The measurements were performed at the experimental temperature of 6 K by utilizing the technique described in detail in Liu et al. [11] Samples similar to those used in BLS measurements (layer thicknesses: Py—5 nm, Pt—4 nm) were placed into a static magnetic field H =520 Oe applied at the angle of 50° with respect to the direction of the current flow. The auto-oscillations of SHNOs were detected by measuring the microwave-frequency component of the voltage generated between the SHNO electrodes due to the anisotropic magnetoresistance. This voltage was amplified by a low-noise microwave amplifier and detected by a microwave spectrum analyser. The microwave signal generated by the SHNO was separated from the synchronizing signal applied at twice the oscillation frequency by utilizing a lowpass filter. Calculations of the current distribution Calculations were performed using a three-dimensional finite-element numerical model of the sample including the Au electrodes and the structured Py/Pt bilayer. The three-dimensional problem based on the Maxwell equations was numerically solved using COMSOL Multiphysics engineering simulation software ( www.comsol.com ). How to cite this article : Demidov, V. E. et al. Synchronization of spin Hall nano-oscillators to external microwave signals. Nat. Commun. 5:3179 doi: 10.1038/ncomms4179 (2014).